Tuning the surface Fermi level onp-type gallium nitride nanowires for efficient overall water splitting Solar water splitting is one of the key steps in artificial photosynthesis for future carbon-neutral, storable and sustainable source of energy. Here we show that one of the major obstacles for achieving efficient and stable overall water splitting over the emerging nanostructured photocatalyst is directly related to the uncontrolled surface charge properties. By tuning the Fermi level on the nonpolar surfaces of gallium nitride nanowire arrays, we demonstrate that the quantum efficiency can be enhanced by more than two orders of magnitude. The internal quantum efficiency and activity on p -type gallium nitride nanowires can reach ~51% and ~4.0 mol hydrogen h −1 g −1 , respectively. The nanowires remain virtually unchanged after over 50,000 μmol gas (hydrogen and oxygen) is produced, which is more than 10,000 times the amount of photocatalyst itself (~4.6 μmol). The essential role of Fermi-level tuning in balancing redox reactions and in enhancing the efficiency and stability is also elucidated. Among the various paths to solar fuel production, the photochemical dissociation of water into its constituent parts, H 2 and O 2, offers the simplest and potentially the most efficient approach; this spontaneous, wireless approach requires virtually zero energy input except sunlight [1] , [2] , [3] , [4] , [5] , [6] , [7] . Recently, nanoscale photocatalysts have been intensively studied that can increase light absorption and charge carrier separation, and therefore enhance the quantum efficiency [8] , [9] , [10] . Fermi-level pinning, however, has been commonly measured on nanowire surfaces [11] . The resulting surface band bending creates an additional energy barrier for charge carrier transport to the photocatalyst–water interface [12] , leading to significantly reduced reaction rate and extremely low efficiency [13] , [14] . To date, the rational synthesis of nanostructured photocatalysts with controlled surface charge properties, that is, tunable surface Fermi level and band bending, has remained a near-universal challenge [9] . Such uncontrolled surface charge properties can further contribute to the photocorrosion and instability of various nanostructures under harsh photocatalysis conditions, severely limiting their practical applications. In this study, we examine the water splitting reaction on the nonpolar surfaces ( m -plane) of GaN nanowire photocatalyst, which may further serve as a new platform for spontaneous water splitting under visible and infrared light irradiation by incorporating indium [15] , [16] . Unique to the nonpolar GaN surfaces is that the occupied surface states are positioned outside of the fundamental energy bandgap and therefore do not create Fermi-level pinning [17] , [18] . The nonpolar surfaces are also highly reactive for spontaneous dissociation of water molecules and possess low energy barrier for proton diffusion [19] , [20] . Owing to the impurity incorporation and/or the presence of any defects, however, an upward (downward) band bending has been commonly measured on n - ( p -) type GaN surfaces [21] , [22] . When n -type GaN surfaces come into contact with water, the upward band bending becomes more severe, as shown in Fig. 1a,b , which can suppress H 2 O reduction reaction. When p -type GaN surfaces are in equilibrium with water, the downward band bending can be enhanced, as shown in Fig. 1c,d , which can limit the H 2 O oxidation reaction. In practice, weakly n -type or nearly intrinsic surfaces are often present on p -doped GaN nanowires, with the Fermi level positioned slightly above the electrochemical potential of water. As a consequence, the downward band bending may actually be reduced when such p -doped GaN nanowires are in equilibrium with water. This provides a distinct opportunity to potentially realize balanced and therefore more efficient redox reactions through tuning the Fermi level on nanowire surfaces. Since water oxidation is often the rate-limiting reaction [20] , [23] , p -doped nanowire photocatalyst can further enhance the overall water splitting efficiency by providing abundant-free holes. To date, however, the achievement of p -doped GaN nanowires with tunable surface Fermi level has remained challenging [24] , [25] ( Supplementary Note 1 ). In this study, we demonstrate that the near-surface band bending of catalyst-free GaN nanowires can be controlled with p -type Mg-dopant incorporation. With optimized surface charge properties, we show that the efficiency of spontaneous overall water splitting may be enhanced by more than two orders of magnitude. 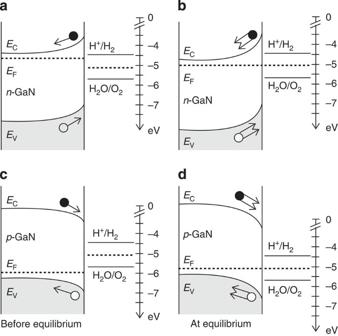Figure 1: Surface band bending ofn- andp-type GaN nanowires. Schematic illustration of the energy band diagram ofn-type GaN nanowire surface (a) before and (b) at equilibrium with water. The upward band bending becomes more severe at equilibrium, which suppresses water reduction reaction. Schematic illustration of the energy band diagram ofp-type GaN nanowire surface (c) before and (d) at equilibrium with water. The downward band bending gets enhanced at equilibrium that suppresses water oxidation reaction. Figure 1: Surface band bending of n - and p -type GaN nanowires. Schematic illustration of the energy band diagram of n -type GaN nanowire surface ( a ) before and ( b ) at equilibrium with water. The upward band bending becomes more severe at equilibrium, which suppresses water reduction reaction. Schematic illustration of the energy band diagram of p -type GaN nanowire surface ( c ) before and ( d ) at equilibrium with water. The downward band bending gets enhanced at equilibrium that suppresses water oxidation reaction. Full size image Structural characterization The GaN nanowires were grown on Si substrate by plasma-assisted molecular beam epitaxy (MBE; Methods section). The Mg-dopant concentration was varied by tuning the Mg effusion cell temperatures ( T Mg ) from 200 to 300 °C. Samples A, B, C, D, E and F correspond to T Mg of 200 °C, 230 °C, 250 °C, 265 °C, 280 °C and 300 °C, respectively. A 45°-tilted scanning electron microscopy (SEM) image of as-grown Mg-doped GaN (denoted as GaN:Mg hereafter) nanowire (sample B) is shown in Fig. 2a (also Supplementary Fig. 1 for SEM images of other samples). The nanowires are ~600 nm in length, ~50–75 nm in diameter and vertically aligned to the substrate. Shown in Fig. 2b is a scanning transmission electron microscopy bright-field (STEM-BF) image, illustrating lattice fringes from defect-free single crystalline nanowire (Methods section). The distance between the two adjacent fringes is about ~0.518 nm that corresponds to the <0001> direction, further confirming that the nanowires are grown along the c axis, with their sidewalls being nonpolar m -planes [26] . Room temperature photoluminescence (PL) measurement clearly shows a single optical emission peak at ~365 nm, corresponding to the bandgap of GaN (3.4 eV) (Methods section and Supplementary Fig. 2 ). For subsequent experiments ~2.8 cm 2 wafer sample was used that corresponds to ~0.387 mg (~4.62 μmol) GaN materials, considering the nanowire fill factors on Si substrate ( Supplementary Fig. 3 ). 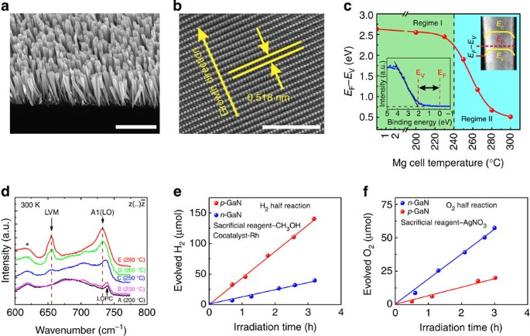Figure 2: Structural characterization and surface charge properties of GaN:Mg nanowires. (a) A 45 ° tilted SEM image of GaN:Mg (sample B) nanowire arrays. Scale bar, 1 μm. (b) STEM-BF lattice image illustrating lattice fringes from defect-free single crystalline GaN:Mg nanowire (sample B). Scale bar, 5 nm. (c)EF−EVfor different GaN:Mg samples determined from ARXPS valence spectrum. The insets illustrateEF−EVon the TEM image of a single nanowire and on an ARXPS valence spectrum.The dotted line separates two regimes, Regime I (n-type surfaces) and Regime II (p-type surfaces). (d) Typical room temperature micro-Raman spectra of GaN nanowires withTMgranging from 200 to 280 °C. Si modes are pointed out with ‘*’ and the dashed lines are guide to the eye. (e) Evolution of H2fromn- (Si-doped) andp-GaN (TMg=230 °C) nanowire arrays in the presence of CH3OH and Rh cocatalyst. Enhanced evolution of H2is observed forp-type GaN nanowires, owing to the presence of downward surface band bending. (f) Evolution of O2fromn- (Si-doped) andp-GaN (TMg=230 °C) nanowire arrays in the presence of AgNO3sacrificial reagent. Enhanced evolution of O2is measured forn-type GaN nanowires, which can be well correlated to the presence of upward surface band bending. The solid lines are guide to the eye. Figure 2: Structural characterization and surface charge properties of GaN:Mg nanowires. ( a ) A 45 ° tilted SEM image of GaN:Mg (sample B) nanowire arrays. Scale bar, 1 μm. ( b ) STEM-BF lattice image illustrating lattice fringes from defect-free single crystalline GaN:Mg nanowire (sample B). Scale bar, 5 nm. ( c ) E F − E V for different GaN:Mg samples determined from ARXPS valence spectrum. The insets illustrate E F − E V on the TEM image of a single nanowire and on an ARXPS valence spectrum.The dotted line separates two regimes, Regime I ( n -type surfaces) and Regime II ( p -type surfaces). ( d ) Typical room temperature micro-Raman spectra of GaN nanowires with T Mg ranging from 200 to 280 °C. Si modes are pointed out with ‘*’ and the dashed lines are guide to the eye. ( e ) Evolution of H 2 from n - (Si-doped) and p -GaN ( T Mg =230 °C) nanowire arrays in the presence of CH 3 OH and Rh cocatalyst. Enhanced evolution of H 2 is observed for p -type GaN nanowires, owing to the presence of downward surface band bending. ( f ) Evolution of O 2 from n - (Si-doped) and p -GaN ( T Mg =230 °C) nanowire arrays in the presence of AgNO 3 sacrificial reagent. Enhanced evolution of O 2 is measured for n -type GaN nanowires, which can be well correlated to the presence of upward surface band bending. The solid lines are guide to the eye. Full size image Near-surface band structure The near-surface band structure of as-grown nanowires can be estimated by measuring the Fermi level ( E F ) relative to the valence band maximum ( E V ). The E F − E V in the near-surface region ( Fig. 2c inset) was measured by recording angle-resolved X-ray photoelectron spectroscopy (ARXPS) valence spectrum ( Fig. 2c inset) from the lateral nonpolar ( m -plane) surfaces of the nanowire (Methods section) [27] . Illustrated in Fig. 2c , the E F − E V is measured to be 2.63 eV for undoped GaN ( T Mg =0 °C), which is similar to the E F − E V (2.6 eV) measured on n -type GaN surfaces by Wu et al. [28] Two distinct regimes are clearly separated with dotted lines. Regime I ( n -type surfaces), wherein the near-surface E F − E V stays nearly constant for T Mg up to 230 °C, which corresponds to the compensation of background n -type dopants by Mg acceptors [29] . Regime II ( p -type surfaces), wherein the near-surface E F − E V decreases drastically with increase in T Mg , is because of the enhancement in free hole concentration in GaN nanowires. In the relatively high bulk-doping regime (samples C–F), variations of E F − E V in the bulk region with increasing Mg cell temperature is estimated to be in the range of tens of meV, which is much smaller than the variation measured in the near-surface region (~2 eV). Consequently, the reduction of E F − E V in the near-surface region, as shown in Fig. 2c , can be directly correlated to the reduction in the downward surface band bending with increasing Mg-dopant incorporation [30] , [31] . In addition, our detailed analysis reveals that variations in the surface band bending have a very small, or negligible dependence on the morphology of GaN nanowires. p -Type doping Variations of the surface charge properties are further probed by micro-Raman measurements at room temperature (Methods section). The evolution of the Raman mode in the range of 600–800 cm −1 with Mg doping is illustrated in Fig. 2d (the complete Raman spectrum is shown in Supplementary Fig. 4 ). For nanowires with the lowest Mg-doping levels (sample A, T Mg =200 °C; and sample B, T Mg =230 °C), a narrow peak at ~741 cm −1 is present, which is attributed to the coupling between the longitudinal optical phonon–plasmon-coupled (LOPC) mode [24] , [32] . The appearance of the LOPC mode is associated with the weakly n -type surfaces for GaN nanowires at relatively low Mg doping (samples A and B), marked as Regime I in Fig. 2c , which can be gradually compensated with further increase in Mg doping/free hole concentration within nanowires. Accordingly, with the increment of Mg-doping level for sample C ( T Mg =250 °C), the LOPC mode gradually shifts to a lower frequency, and also its intensity becomes stronger because of the reduced coupling effect between the LO phonon and electron plasmon. With further increment of the Mg-doping level in sample D ( T Mg =265 °C), the frequency of the LOPC mode shifts to ~733 cm −1 (the original frequency of the pure uncoupled A 1 (LO) mode). It indicates that the coupling between the LO phonon and electron plasma is completely suppressed in more heavily doped GaN nanowires, which is consistent with the measured surface type (weakly p -type, Regime II shown in Fig. 2c ). The presence of p -type surfaces, evidenced by both the ARXPS and the pure uncoupled A 1 (LO) mode, is also well correlated with the appearance of an extra mode at 655 cm −1 in sample C ( T Mg =250 °C). Such a foreign Raman mode is attributed to the local vibrational modes related to Mg impurity (Mg–N bond) [33] . Its intensity is directly proportional to the free hole concentration ( Supplementary Fig. 5 ) [28] and becomes stronger with further increment of Mg-doping level in samples D ( T Mg =265 °C) and E ( T Mg =280 °C). H 2 and O 2 half reactions The tunable surface Fermi level and the engineered surface charge properties are essential to achieve controlled redox reactions. To demonstrate this hypothesis, H 2 and O 2 half reactions in the presence of respective sacrificial reagents were first performed using both n - (Si-doped) and p -type GaN nanowire arrays (Methods section). Figure 2e shows the evolution of H 2 from n - and p -type (sample B, T Mg =230 °C) GaN nanowire arrays in the presence of Methanol (CH 3 OH) and Rhodium (Rh) cocatalyst. The H 2 generation rate of p -type GaN nanowire is significantly higher than conventional n -type GaN nanowires, owing to the downward band bending at the surface of p -type GaN ( Fig. 1c ). In contrast, as shown in Fig. 2f , the activity for O 2 generation is significantly enhanced on n -type GaN nanowires with an upward surface band bending ( Fig. 1a ). For overall water splitting and stoichiometric evolution of H 2 and O 2 ; however, both oxidation and reduction reaction need to proceed simultaneously [4] . The presence of any upward or downward band bending will create additional uphill barriers for one of these two reactions, and therefore severely limit overall water splitting efficiency. Since the downward band bending reduces with increase in T Mg in the p -type surface regime ( Fig. 2c , Regime II), efficient carrier transport and therefore high photocatalytic activity is expected for optimized p -doping levels. Rh/Cr 2 O 3 cocatalyst To further enhance the charge carrier extraction and provide more active sites for gas generation, Rh/Chromium-oxide (Cr 2 O 3 ) cocatalyst nanoparticles are deposited on all the samples (A-F) using photodeposition process from liquid precursors (Methods section) [14] . 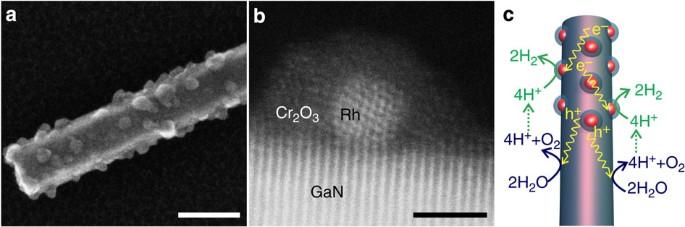Figure 3: TEM characterization of core-shell Rh/Cr2O3nanoparticles on GaN nanowire. (a) Low-magnification STEM-SE image. Scale bar, 50 nm. (b) STEM-HAADF image of Rh/Cr2O3nanoparticle-decorated GaN:Mg nanowire. Scale bar, 2 nm. Crystalline Rh core and amorphous Cr2O3shell are clearly observed. (c) Schematic of Rh/Cr2O3-decorated GaN nanowire and the water splitting mechanism. Figure 3 shows (a) a low magnification STEM secondary electron (SE) image; and (b) a STEM-high-angle annular dark-field (HAADF) image of Rh/Cr 2 O 3 nanoparticle-decorated GaN nanowire. These images reveal that the Rh/Cr 2 O 3 nanoparticles are successfully deposited in the form of core-shell nanostructures on GaN nanowire surfaces. In addition, the Rh core and GaN nanowire show single crystalline structure. The presence of metallic Rh, mixed Rh-Cr oxide, and Cr 2 O 3 nanoparticles was further confirmed by ARXPS ( Supplementary Note 2 and Supplementary Fig. 6 ). The Rh core facilitates carrier migration to the nanowire surface and reduces the activation energy required for gas evolution. The Cr 2 O 3 shell suppresses the back reaction to form H 2 O from H 2 and O 2 on the Rh core [15] . The role of cocatalyst was further elucidated by control-experiments ( Supplementary Note 3 and Supplementary Fig. 7 ). Figure 3c shows a schematic of the core-shell Rh/Cr 2 O 3 nanoparticle deposited GaN nanowire for overall water splitting, illustrating the reaction mechanism on the nonpolar surfaces of GaN nanowires. Figure 3: TEM characterization of core-shell Rh/Cr 2 O 3 nanoparticles on GaN nanowire. ( a ) Low-magnification STEM-SE image. Scale bar, 50 nm. ( b ) STEM-HAADF image of Rh/Cr 2 O 3 nanoparticle-decorated GaN:Mg nanowire. Scale bar, 2 nm. Crystalline Rh core and amorphous Cr 2 O 3 shell are clearly observed. ( c ) Schematic of Rh/Cr 2 O 3 -decorated GaN nanowire and the water splitting mechanism. Full size image Overall pure water splitting The Rh/Cr 2 O 3 nanoparticle-decorated GaN nanowires with different Mg-doping levels were subsequently used for overall pure (pH~7.0) water splitting under 300 W full arc Xenon lamp irradiation. 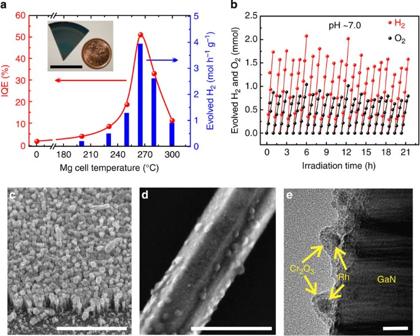Figure 4: Overall water splitting and stability of GaN:Mg nanowires. (a) H2evolution rate and internal quantum efficiency (IQE) for different GaN:Mg samples in overall pure water splitting. Reactions were performed using ~0.387 mg GaN nanowire catalyst in pure water under illumination of a Xenon lamp (300 W). The sample size is shown in the inset. Scale bar 2 cm. (b) Repeated cycles of overall pure water splitting for GaN:Mg: 265 °C (sample D), showing the stability of the nanowires. (c) A bird’s-eye view SEM image of the GaN nanowire arrays after ~22 h of overall water splitting. Scale bar, 2 μm. (d) Low-magnification STEM-SE image of a single nanowire after overall water splitting reaction for ~22 h. Scale bar, 100 nm. (e) High-resolution BF TEM image after reaction, showing the stability of core-shell Rh/Cr2O3nanoparticles and GaN nanowire. Scale bar, 10 nm. The solid lines are guide to the eye. Figure 4a shows the H 2 evolution rates for different GaN:Mg nanowire samples, which were derived from 6 h overall water splitting reaction on each sample. It is seen that the H 2 evolution rate first shows a marked increase with Mg cell temperature. Under relatively low doping levels (samples A and B), the photocatalytic activity is low, which is directly correlated to the very large downward surface band bending ( Fig. 1d ), because of the weakly n -type surface-nature as revealed from ARXPS and micro-Raman analysis ( Fig. 2c , Regime I, and Fig. 2d ). Markedly enhanced overall water splitting performance was measured for sample D ( T Mg =265 °C), and the H 2 evolution rate was nearly 4 mol h −1 g −1 , which is more than two orders of magnitude higher, compared with the nominally undoped GaN nanowires [14] . This drastic improvement can be well explained by the p -type surfaces with significantly reduced downward band bending ( Fig. 2c , Regime II, and Fig. 2d ), which may become relatively flat in aqueous solution, thereby enabling balanced and much more efficient redox reactions. For samples E ( T Mg =280 °C) and F ( T Mg =300 °C), however, the activity shows a decreasing trend with increase in Mg cell temperature, which is likely to be related to the degradation of GaN nanowire crystalline quality at very high Mg-doping level [24] , [34] , [35] ( Supplementary Note 4 ). For optimum Mg-doping concentration (sample D), the apparent quantum efficiency can reach ~18% ( Supplementary Note 5 ). The internal quantum efficiency, as shown in Fig. 4a , is also derived for different Mg-doped samples under ~200–365 nm wavelength ( Supplementary Note 5 ). It can reach ~51% for GaN nanowires with optimum surface band bending (sample D), which is the highest value reported for spontaneous overall water splitting under any broadband light irradiation to our knowledge [4] , [36] , [37] . Figure 4: Overall water splitting and stability of GaN:Mg nanowires. ( a ) H 2 evolution rate and internal quantum efficiency (IQE) for different GaN:Mg samples in overall pure water splitting. Reactions were performed using ~0.387 mg GaN nanowire catalyst in pure water under illumination of a Xenon lamp (300 W). The sample size is shown in the inset. Scale bar 2 cm. ( b ) Repeated cycles of overall pure water splitting for GaN:Mg: 265 °C (sample D), showing the stability of the nanowires. ( c ) A bird’s-eye view SEM image of the GaN nanowire arrays after ~22 h of overall water splitting. Scale bar, 2 μm. ( d ) Low-magnification STEM-SE image of a single nanowire after overall water splitting reaction for ~22 h. Scale bar, 100 nm. ( e ) High-resolution BF TEM image after reaction, showing the stability of core-shell Rh/Cr 2 O 3 nanoparticles and GaN nanowire. Scale bar, 10 nm. The solid lines are guide to the eye. Full size image In order to reveal the stability of the GaN photocatalyst, repeated experiments were performed using the same sample. Figure 4b shows the evolution of H 2 and O 2 as a function of irradiation time for the optimized GaN:Mg (sample D) in pure water. No sacrificial reagents were added in the reaction. The rates of H 2 and O 2 evolution were ~1,525 and ~763 μmol h −1 , respectively. The H 2 /O 2 ratio is nearly 2:1, indicating a balanced redox reaction of water on the nanowire photocatalyst. Visible bubbles were clearly observed from the sample surface upon irradiation ( Supplementary Movie 1 ). The turnover number, defined as the ratio of the total amount of gas evolved (50,428 μmol) to GaN catalyst (4.62 μmol), exceeded ~10,915 during the course of ~22 h of reaction. Repeated experiments on the same sample did not show any degradation of the photocatalytic activity, demonstrating excellent stability of the Mg-doped GaN nanowires. The turnover number in terms of the ratio of the rate of H 2 molecules formed to the rate of absorbed photons is also plotted as a function of time ( Supplementary Fig. 8 ), further confirming excellent stability of the nanowire photocatalyst. The slight variations in H 2 and O 2 evolution observed for different cycles are attributed to the variations in alignment between the light source and the sample surface. Figure 4c shows a SEM image of the nanowire arrays (sample D) after overall water splitting for ~22 h. The nanowires remain stable during the course of the reaction. A low-magnification STEM-SE image of a single nanowire, as shown in Fig. 4d , further confirms that the cocatalyst nanoparticle-decorated GaN nanowire were not etched during the course of reaction, which can be partially attributed to the surface free-holes of Mg-doped GaN that can prevent the catalyst from photocorrosion caused by oxidation [38] . The core-shell Rh/Cr 2 O 3 nanoparticles are also stable in photocatalytic environment, as shown in the BF TEM image in Fig. 4e . In summary, we have demonstrated that by tuning the surface Fermi level through controlled Mg-dopant incorporation, the quantum efficiency for spontaneous pure water splitting on GaN nanowire arrays can be enhanced by nearly two orders of magnitude, and the activity can reach ~4.0 mol hydrogen h −1 g −1 , which is much higher than previously reported photocatalyst materials [36] . Future work includes the demonstration of high efficiency and stable overall water splitting under visible and infrared light irradiation by engineering the surface charge properties of InGaN nanowires. MBE growth Catalyst-free vertically aligned GaN nanowires were grown on n -Si (111) substrate by radio frequency plasma-assisted MBE under nitrogen rich conditions. Thermal effusion cells were used for Ga and Mg. The native oxide on Si substrate was etched with 10% hydrofluoric acid (HF) for 30 s before loading into the MBE chamber. The growth parameters include a growth temperature of ~750 °C, nitrogen flow rate of 1.0 standard cubic centimeters per minute (sccm), a forward plasma power of ~350 W and a Ga beam equivalent pressure of ~6 × 10 −8 Torr. The growth duration was ~4 h. The Mg beam equivalent pressure was varied from ~0.2 × 10 −10 to ~1.5 × 10 −9 Torr for Mg cell temperatures from 200 to 300 °C. Note that, because of the presence of conduction and valence band offsets at the GaN/Si interface, the photoexcited carriers in Si substrate do not take part in the photochemical reaction [15] . Transmission electron microscopy A CM200 microscope with an accelerating voltage of 200 kV was used to obtain BF TEM images. For STEM-SE and STEM-HAADF imaging, a Hitachi HD2700 Cs-corrected STEM with a cold-field emission emitter operated at 200 kV and with an electron beam diameter of ~0.1 nm was used. PL measurement A 325-nm He–Cd laser (Kimmon Koha) was used as the excitation source for the PL measurement of the nanowire heterostructure. The PL was spectrally resolved by a high-resolution spectrometer and detected by a photomultiplier tube. Room temperature PL spectrum of GaN:Mg nanowires, with Mg effusion cell temperature of 230 °C, is shown in Supplementary Fig. 2 . Micro-Raman measurement Micro-Raman measurements were carried out at room temperature with an external 488 nm Argon-ion laser through a × 100 objective with a numerical aperture ~0.9. The focused laser spot size was ~1 μm and the estimated incident power was ~40 mW. The Raman signal was collected by a Synapse CCD air-cooled detector. The incident laser was parallel with the hexagonal c axis of the nanowires, and the laser light was scattered without polarization analysis ( z(..)z direction). Photocatalytic reaction The photocatalytic reaction was performed in a Pyrex chamber with a quartz lid. A 300-W Xenon lamp (Cermax, PE300BUV) was used as an outer irradiation source. Distilled water (pH ~7.0) was used for the pure water splitting reaction. The H 2 half reaction was performed in the presence of CH 3 OH (20 vol.%) as electron donor and Rh nanoparticles as cocatalyst. For O 2 half reaction, AgNO 3 (0.1 M) was used as electron acceptor. The water was purged with Ar for 30 min before each experiment. The chamber was then evacuated. The gases produced from the reaction were sampled using a vacuum tight syringe. A gas chromatograph (Shimadzu GC-8A) equipped with thermal conductivity detector and high-purity Ar carrier gas was used to analyse the reaction-evolved gases. The experimental error in the evolution of H 2 and O 2 is estimated to be ~10%, which is ascribed to the manual sampling of the gases. Photodeposition of Rh/Cr 2 O 3 core-shell nanoparticles The deposition of Rh/Cr 2 O 3 core-shell nanoparticles on the GaN nanowires was performed following a two-step photodeposition process. First, 2 μl of 0.2 M sodium hexachlororhodate(III) (Na 3 RhCl 6 , Sigma-Aldrich), 12 ml of CH 3 OH and 60 ml of distilled water (purged with pure Argon for 30 min) were placed in a 460 ml Pyrex chamber (Kimble Chase) with quartz lid. The GaN nanowire photocatalyst (on Si substrate) was placed in the Pyrex chamber using a homemade polytetrafluoroethylene holder. The chamber was then pumped down for 10 min and subsequently irradiated for 30 min using 300 W Xenon lamp (Cermax, PE300BUV) for photo-assisted deposition of Rh nanoparticles. The sample was dried in air for a few minutes. In the second step, the Cr 2 O 3 was deposited following the above-mentioned procedure by 2 μl of 0.2 M potassium chromate (K 2 CrO 4 , Sigma-Aldrich) as precursor. Angle-resolved X-ray photoelectron spectroscopy The monochromatic Al-Kα X-ray source (h υ =1486.6 eV) was placed 60° with the surface normal to excite the nonpolar surfaces of GaN nanowire arrays. The high-resolution XPS spectra were obtained using an X-ray beam size of 400 μm, pass energy of 50 eV and a step size of 0.1 eV. Individual peak fitting was performed using convolution of Lorentzian and Gaussian line shapes (L/G=30%) with Avantage software (Thermo Scientific). The binding energies were calibrated with both Au-4f peak (84.0 eV) and C-1s peak (285.0 eV) before each experiment. The E F − E V was estimated from ARXPS valence spectrum with linear extrapolation of the valence band leading edge and the baseline as shown in the inset of Fig. 2c . The intersection between these two lines indicates the position of surface valence band with respect to the surface Fermi level (binding energy=0 eV) [27] . How to cite this article: Kibria, M. G. et al. Tuning the surface Fermi level on p -type gallium nitride nanowires for efficient overall water splitting. Nat. Commun. 5:3825 doi: 10.1038/ncomms4825 (2014).